Highly selective single and multiple deuteration of unactivated C(sp3)-H bonds Selective deuteration of unactivated C(sp 3 )-H bonds is a highly attractive but challenging subject of research in pharmaceutical chemistry, material science and synthetic chemistry. Reported herein is a practical, highly selective and economical efficient hydrogen/deuterium (H/D) exchange of unactivated C(sp 3 )-H bonds by synergistic photocatalysis and hydrogen atom transfer (HAT) catalysis. With the easily prepared PMP-substituted amides as nitrogen-centered radical precursors, a wide range of structurally diverse amides can undergo predictable radical H/D exchange smoothly with inexpensive D 2 O as the sole deuterium source, giving rise to the distal tertiary, secondary and primary C(sp 3 )-H bonds selectively deuterated products in yields of up to 99% and excellent D-incorporations. In addition to precise monodeuteration, this strategy can also achieve multideuteration of the substrates contain more than one remote C(sp 3 )-H bond, which opens a method to address multi-functionalization of distal unactivated C(sp 3 )–H bonds. The precise deuterium labeling technique is of significant value in the investigation of kinetic isotopic effects [1] , [2] , the discovery of pharmaceutical drugs [3] , [4] , [5] , [6] , and material modifications [7] as well as biochemical techniques [8] , [9] (Fig. 1a ). In recent decades, the synthesis of deuterated molecules has attracted much attention from organic chemists [10] , [11] , [12] , [13] , [14] , [15] , [16] , [17] , [18] , [19] , [20] , [21] , [22] , [23] , [24] , [25] , [26] , [27] , [28] , [29] . For instance, our group has developed a practical deoxygenative deuteration of carboxylic acids for the synthesis of D-labeled aldehydes using synergistic catalysis [16] . Among various reliable synthetic methods for deuterium incorporation, the radical hydrogen−deuterium (H/D) exchange strategy of C(sp 3 )-H bonds is one of the most practical and atom-economical methods due to the mild reaction conditions and the excellent functional group compatibility. In 2017 for example, MacMillan et al. [30] developed an elegant photoredox-catalyzed H/D exchange of α-amino C(sp 3 )–H bonds, and in 2020, Wu et al. reported a visible-light-driven H/D exchange of hydridic C(sp 3 )–H bonds with tetrabutylammonium decatungstate (TBADT) [31] . Notwithstanding these efforts, radical H/D exchange of unactivated C(sp 3 )-H bonds remains highly challenging due to the stronger bond dissociation energy (BDE) of unactivated C(sp 3 )-H bonds compared with C(sp 3 )-H moieties adjacent to an aryl ring or a heteroatom (Fig. 1b ). Fig. 1: Project background and design plan for radical deuteration of unactivated C(sp 3 ) bonds. a The significance of deuterated compounds. b The BDE of different C(sp 3 )-H bonds and stability of related alkyl radicals. c Previous work on N-X bonds cleavage induced deuteration of remote C(sp 3 )-H bonds. d This work: Tunable H/D exchange of single or multiple unactivated C(sp 3 )-H bonds. Full size image Very recently, Studer and coworkers [32] reported an interesting radical monodeuteration of remote unactivated C(sp 3 )-H bonds via 1,5-hydrogen atom transfer (HAT) induced by a nitrogen-centered radical, which is generated in-situ using a stoichiometric of thiol (RSH) in the presence of AIBN at 85 °C (Fig. 1c ). This is a powerful method, but the preinstallation of an allylsulfonyl moiety on the nitrogen atom is crucial to successful initiation of the radical rearrangement to generate the N-centered radical and produce 1 equivalent of SO 2 and allylsulfides as the concomitant products. Thus we questioned if the more challenging free N-H contained amides are competent substrates for radical H/D exchange of remote C(sp 3 )-H bonds through proton-coupled electron transfer (PCET) [33] , [34] , [35] , [36] process. The key challenges to such reactions stem from concerns that the single electron oxidation of strong N-H bonds (100~110 kcal mol −1 ) [37] , [38] and the acidic protons in N-H moiety would prevent a high deuterium incorporation from D 2 O. Herein, we develop a highly selective and efficient hydrogen/deuterium (H/D) exchange of unactivated C(sp 3 )-H bonds by using D 2 O as commercially cheap deuterium source, delivering a wide range of remote tertiary, secondary and primary C(sp 3 )-H bonds deuterated amides in high yields and D-incorporations. Moreover, with this protocol, the precise radical H/D exchange of multiple remote C(sp 3 )-H bonds also has been realized (Fig. 1d ). Substrate design We first performed DFT calculations to estimate the BDEs of N-H bonds with different substituents and the singly occupied molecular orbital (SOMO) energies of the corresponding nitrogen radicals. Interestingly, it was found that different amides have different N-H BDEs and different SOMO energies of nitrogen-centered radicals, which indicates a possibility with which to tune the reactivity towards the PCET and 1,5-HAT processes by synergistic photoredox catalysis. As shown in Fig. 1d , the N-H bond in the PMP-substituted amide ( 1c ) has a moderate BDE (~104 kcal mol −1 ) while the corresponding nitrogen-centered radical has the highest SOMO energy (−7.58 eV). According to the polarity-matching rule, this might favor a fast 1,5-HAT process of unactivated C(sp 3 )-H bonds. 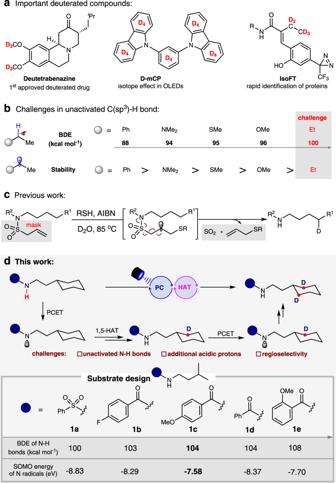Fig. 1: Project background and design plan for radical deuteration of unactivated C(sp3) bonds. aThe significance of deuterated compounds.bThe BDE of different C(sp3)-H bonds and stability of related alkyl radicals.cPrevious work on N-X bonds cleavage induced deuteration of remote C(sp3)-H bonds.dThis work: Tunable H/D exchange of single or multiple unactivated C(sp3)-H bonds. Reaction optimization Experimental results have shown that the amide 1c is the most efficient substrate, and can afford the desired D-labeled product ( 3c ) in 85% isolated yield with 0.97 D by using D 2 O as the sole D-source (Table 1 , entry 1). It was found that the optimal reaction conditions include Ir III (1 mol%) as the photocatalyst, Bu 4 NOP(O)(OBu) 2 (5 mol%) as base, 2a (10 mol%) as HAT catalyst and chlorobenzene (PhCl) as solvent. Other substituted amides ( 1a , 1b , 1d and 1e ) were also examined under these conditions (entries 2–5) but the D-incorporations of benzenesulfonamide ( 1a ), 4-fluorobenzamide ( 1b ), benzamide( 1d ) and 2-methoxyphenyl-substituted amide ( 1e ) were found to be significantly lower (<0.30 D), this might be caused by the mismatched SOMO energy or strong DBE of the N-H bond. Importantly, base optimization experiments illustrated the unique role of Bu 4 NOP(O)(OBu) 2 (entries 6 and 7). We envisioned that the phosphate base would accelerate the PCET process by the hydrogen bonding between the amide N-H and the phosphate anion [39] . In addition to the HAT catalyst 2a , other thiols ( 2b and 2c) are also good HAT catalysts, which can furnish the target product in good yield with slightly decreased D-incorporation (entries 8 and 9, 0.92 D and 0.95 D respectively). The use of other solvents, such as PhCF 3 or toluene (entries 10 and 11), can deliver the products in satisfactory results (>95% yields with 0.92 D). Table 1 Optimization of reaction conditions a . Full size table Substrate scope To evaluate the functional group generality of this H/D exchange strategy, a variety of structurally diverse amides were subjected to this protocol. 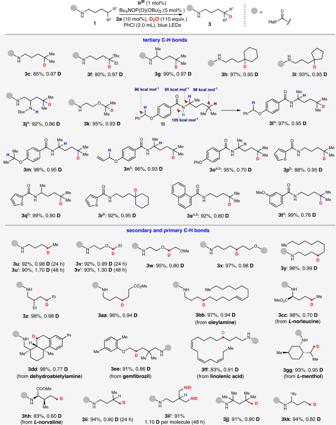Fig. 2: Scope of the radical H/D exchange of C(sp3)-H bonds. Reaction conditions: IrIII(1 mol%), Bu4NOP(O)(OBu)2(5 mol%),2a(10 mol%), amide1(0.1 mmol), D2O (110 equiv., 0.2 mL), PhCl (2.0 mL), blue LEDs, 24 h, ambient temperature (with a fan to cool), in argon atmosphere. Isolated yields are shown and the deuterium incorporation ratio was determined by1H NMR spectroscopy. PMP = 4-methoxyphenyl.a48 h.b2c(10 mol%) instead of2a. In general, the tertiary, secondary and primary C(sp 3 )-H bonds of those amides were smoothly converted to C(sp 3 )-D bonds ( 3c , 3f – 3kk ) in excellent yields and D-incorporations. As shown in Fig. 2 , we first investigated the compatibility of PMP-substituted amides with a remote tertiary C-H bond ( 3c , 3f – 3k ). The H/D exchange of amides containing five- or six-membered carbocycles ( 3 h , 3i ), or an oxygen atom ( 3k ) worked efficiently (>90% yield, >0.90 D). When the amide ( 1j ) has an acidic hydrogen (BocN-H), the D-incorporation of corresponding product ( 3j ) was decreased slightly (0.86 D). Apart from PMP-substituted amides, other diverse benzamide derivatives ( 1l – 1t ) were deuterated smoothly as well with a moderate to good D-incorporation of 0.70–0.95 D ( 3l – 3t ). More significantly, the chemoselectivity of this H/D exchange was found to be promising ( 3l – 3o ). Hydridic C(sp 3 )–H bonds such as those in benzylic, allylic, α-amino or α-oxy positions in amides remain intact during radical H/D exchange even though the relevant BDEs are much lower than those of remote unactivated C(sp 3 )–H bonds. Achieving this result by other H/D exchange strategy [31] is very difficult and further demonstrates the excellent regioselectivity of the 1,5-HAT process. Fig. 2: Scope of the radical H/D exchange of C(sp 3 )-H bonds. Reaction conditions: Ir III (1 mol%), Bu 4 NOP(O)(OBu) 2 (5 mol%), 2a (10 mol%), amide 1 (0.1 mmol), D 2 O (110 equiv., 0.2 mL), PhCl (2.0 mL), blue LEDs, 24 h, ambient temperature (with a fan to cool), in argon atmosphere. Isolated yields are shown and the deuterium incorporation ratio was determined by 1 H NMR spectroscopy. PMP = 4-methoxyphenyl. a 48 h. b 2c (10 mol%) instead of 2a . Full size image Compared with tertiary C(sp 3 )-H bonds, the 1,5-HAT of primary and secondary C(sp 3 )-H bonds is more challenging due to the higher BDEs and lower stability of carbon-centered radicals [40] , [41] , [42] , [43] , [44] . Despite this, the deuteration of the secondary C(sp 3 )-H bonds ( 3u – 3ff ) proceeded perfectly (>95% yields, >0.70 D) with good functional group (-OMe, -COOMe and alkenyl) tolerance. And primary C(sp 3 )-H bonds are also suitable for this protocol, the remote deuterated products ( 3gg-3kk ) were obtained in good yields with acceptable D-incorporations (0.60–0.95 D). Moreover, the derivatives of some complex molecules, such as oleylamine, L -norleucine, dehydroabietylamine, gemfibrozil, linolenic acid, L -menthol, L -norvaline, can undergo this radical H/D exchange smoothly to give the products ( 3bb – 3hh ) with moderate to good D-incorporations. Furthermore, we found that the multiple deuteration products 3 u’ , 3 v’ and 3ii’ (a mixture of mono- and di-deuterated compound) of secondary or primary C(sp 3 )-H bonds can be obtained by prolonging the reaction time from 24 h to 48 h. Inspired by the di-deuteration of 1ii , we wondered that beyond the precise deuteration of one remote C(sp 3 )-H bond, if this 1,5-HAT strategy can achieve the di-deuteration of two remote unactivated C-H bonds. Delightfully, our method successfully realized the multideuteration when the substrate contains more than one remote C(sp 3 )-H bond (Fig. 3 ), a result that is difficult to achieve with previous method [32] . To investigate the practicality of this finding, a wide range of amides with six-membered rings were examined. Structures containing cyclohexane ( 4a , 4c and 4d ), tetrahydropyran ( 4b ), hexahydropiperidine ( 4e , 4 f ) and morpholine ( 4 g ) were successfully multideuterated with 1.20–2.15 D per molecule. The gem-difluoride group ( 4d , 89% yield, 1.40 D per molecule), the ester group ( 4c , 86% yield, 1.20 D per molecule) were entirely compatible. Additionally, the adamantyl ( 4 h , 92% yield, 1.84 D per molecule), cyclopentyl ( 4i , 96% yield, 2.50 D per molecule) and tetrahydropyrrolyl ( 4j , 94% yield, 1.67 D per molecule) groups performed excellently. Besides cyclic compounds, the acyclic structures including both secondary and primary C(sp 3 )-H bonds were converted to the corresponding multi-deuterated products ( 4k-4o ) in excellent yield (86%-97%) and satisfactory D-incorporation (1.50–4.00 D per molecule). This unprecedented process provides an opportunity for the multi-functionalization of distal unactivated C(sp 3 )–H bonds. Fig. 3: Multi-deuteration of C(sp 3 )-H bonds. Reaction conditions: Ir III (1 mol%), Bu 4 NOP(O)(OBu) 2 (5 mol%), 2a (10 mol%), 1 (0.1 mmol), D 2 O (110 equiv., 0.2 mL), PhCl (2.0 mL), blue LEDs, 24 h, ambient temperature (with a fan to cool), in argon atmosphere. Isolated yields are shown and the deuterium incorporation ratio was determined by 1 H NMR spectroscopy. a 12 h. b 48 h. Full size image Synthetic application As shown in Fig. 4 , when the remote deuteration reaction of 1 u was scaled-up to 5.0 mmol, 3 u was obtained with quantitative yield and satisfying D-incorporation (0.98 D). There are some promising synthetic potentials of this deuterated amide product ( 3 u ), which is a versatile substrate for downstream transformations to deliver the secondary amine ( 5 ) and tertiary amide ( 6 ) in excellent yields. Additionally, the amide group in 3 u can be esteemed as a directing group for transition-metal-catalyzed C − H bond functionalization. For example, rhodium-catalyzed C-H activation of 3 u can react with diphenyl acetylene successfully to generate the oxidative cycloaddition product ( 7 ). A photoredox/nickel dual catalyzed C(sp 2 )-C(sp 3 ) coupling of 3 u with bromobenzene to afford product ( 8 ) further demonstrated its synthetic robustness of the deuterated amide. Fig. 4: Synthetic application. a 5 mmol scale-up experiment. b Downstream synthetic transformations and please see Supplementary Information for reaction conditions. Full size image Mechanism proposal As the use of strong base KO t Bu failed in this deuteration reaction, we exclude the deprotonation-electron transfer pathway [33] and a plausible mechanism based on our previous work on synergistic catalyzed deuteration [16] , [17] , [45] , [46] , [47] , [48] , [49] , [50] , [51] , [52] , [53] is proposed in Fig. 5 . We anticipate that firstly, a non-covalent complex will be formed between the Ir III photocatalyst and Bu 4 NOP(O)(OBu) 2 [54] . The resulting Ir III -complex formed in-situ is excited to Ir III * by visible light and meanwhile a hydrogen bond is formed from (BuO) 2 PO 2 − and the amide N − H of substrate ( 1c ), thus triggering the PCET process [39] to generate the nitrogen radical ( 9 ). Then the hydrogen atom of the remote C(sp 3 )-H is transferred to the N-radical and a carbon-centered radical ( 11 ) is produced via a six-membered ring intermediate ( 10 ). In a HAT catalytic cycle analogous to our previous work [16] , [17] , RSD is generated in-situ from RSH and excess D 2 O as a result of the distinction in the pK a values. 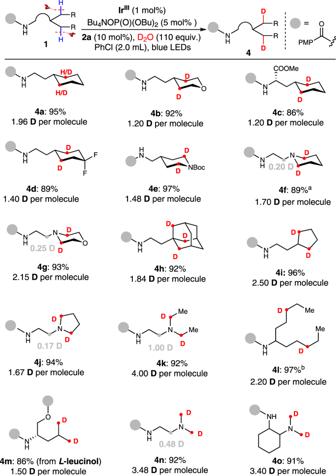Fig. 3: Multi-deuteration of C(sp3)-H bonds. Reaction conditions: IrIII(1 mol%), Bu4NOP(O)(OBu)2(5 mol%),2a(10 mol%),1(0.1 mmol), D2O (110 equiv., 0.2 mL), PhCl (2.0 mL), blue LEDs, 24 h, ambient temperature (with a fan to cool), in argon atmosphere. Isolated yields are shown and the deuterium incorporation ratio was determined by1H NMR spectroscopy.a12 h.b48 h. Subsequently, the nucleophilic alkyl radical ( 11 ) undergoes deuterium atom transfer (DAT) from RS-D, furnishing the desired product ( 3c ). 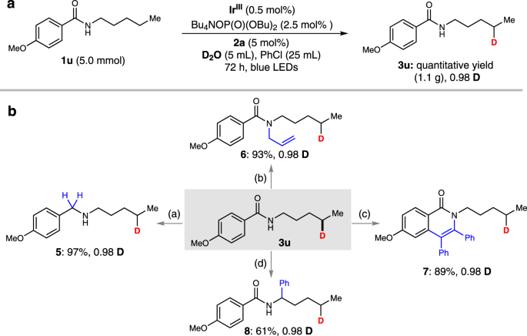Fig. 4: Synthetic application. a5 mmol scale-up experiment.bDownstream synthetic transformations and please see Supplementary Information for reaction conditions. 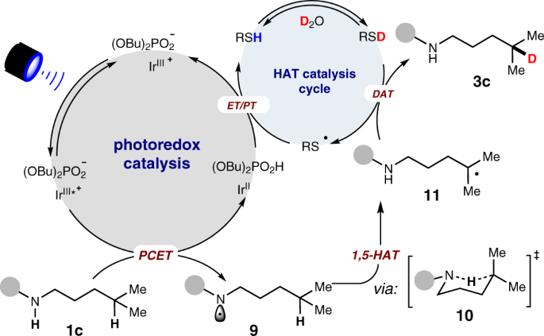Fig. 5: Mechanism proposal. Proposed mechanism for this synergistic catalyzed remote C-H bond deuteration. The resulting electrophilic thiyl radical is readily reduced by Ir II to thiol anion and also complete the photocatalytic cycle [39] , and this is followed by a proton transfer from Bu 4 NOPO 2 H (pKa ≈ 12 in MeCN) [55] to regenerate RSH (pK a ≈ 21 in MeCN for PhSH) [56] , [57] . Fig. 5: Mechanism proposal. Proposed mechanism for this synergistic catalyzed remote C-H bond deuteration. Full size image We have developed a highly selective, economic and practical H/D exchange protocol of remote unactivated C(sp 3 )-H bonds with D 2 O as cheap deuderium source by utilzing a synergistic photoredox catalysis and organocatalysis system. With the DFT calculation optimized free N-H contained amides as N-radical precusor to abstract the remote hydrogen, a wide range of remote tertiary, secondary and primary C(sp 3 )-H bonds can be smoothly converted to the corresponding C-D bonds in excellent yields (up to 99%) and high levels of D-incorporation. This protocol can also achieve tunable multideuteration of substrates containing more than one remote C(sp 3 )-H sites, which represents an significant step-forward in 1,5-HAT-induced multi-functionaztion. This report is an important advance in the controllable synthesis of monodeuterated and multideuterated compounds. General procedure for deuteration A screw cap dram vial was charged with Ir III (1.1 mg, 1 mol%), tetrabutylammonium dibutyl phosphate (2.3 mg, 5 mol%), thiol catalyst 2a (2.8 mg, 10 mol%) or 2c (2.4 mg, 10 mol%), amide (0.1 mmol, 1 equiv), then the vial was delivered to glove box, PhCl (2.0 mL) and D 2 O (0.2 mL) were added. The vial was stirred under the irradiation of blue LEDs at room temperature for the indicated time. After the reaction was finished, the reaction mixture was extracted by ethyl acetate, dried by anhydrous Na 2 SO 4 , filtered and collected the organic layer. The organic solvent was removed under the reduced pressure. The residue was purified by column chromatography on silica gel to obtain the desired products.